Stereospecific ring expansion from orthocyclophanes with central chirality to metacyclophanes with planar chirality Carbon–carbon bonds constitute the major framework of organic molecules and carbon–hydrogen bonds are abundant in their peripheries. Such nonpolar σ-bonds are thermodynamically stable and kinetically inert in general. Nonetheless, selective activation of those ubiquitous bonds may offer a straightforward method to construct and/or functionalize organic skeletons. Herein we describe ring expansion from orthocyclophanes to metacyclophanes occurring upon sequential action of light and a metal catalyst. Formally, specific non-strained carbon–hydrogen and carbon–carbon bonds are cleaved and exchanged without elimination of any leaving groups. Notably, the product is energetically uphill from the starting material, but the endergonic photocyclization step makes it possible to drive the transformation forward. The ring expansion is extended to the stereospecific synthesis of metacyclophanes possessing planar chirality, during which central chirality on a tertiary carbon is transferred to planar chirality. The number of functional groups that can be transformed by transition metal catalysis has been considerably expanded. Carbon–carbon (C–C) [1] , [2] , [3] , [4] , [5] , [6] , [7] , [8] , [9] , [10] , [11] , [12] , [13] , [14] , [15] and carbon–hydrogen (C–H) bonds [16] , [17] , [18] , [19] , [20] , [21] , [22] , [23] , [24] , [25] , which are ubiquitous in organic compounds, are intrinsically difficult to activate owing to their thermodynamic stability as well as their kinetic inertness. Selective transformation of such nonpolar σ-bonds has provided a challenge that has motivated and inspired chemists to seek ways to activate these bonds over the past two decades. Metacyclophanes are cyclic compounds that have a central arene unit with its 1,3-positions connected through an ansa chain [26] . The arene unit can rapidly flip in many cases, but when the flipping is hindered, metacyclophanes can gain stable planar chirality. Such an intriguing chiral metacyclophane unit is found in various natural products like galeon and vancomycin [27] . Chiral metacyclophanes also constitute a key structural component of some pharmaceuticals [28] , [29] and supramolecular host materials that accept small molecules [30] , [31] , [32] . Consequently, the development of methods to stereoselectively construct chiral metacyclophane skeletons has been of growing interest [33] , [34] , [35] , [36] , [37] , [38] . We herein describe a sequential process to expand orthocyclophanes 1 into their more strained constitutional isomers, metacyclophanes 2 ( Fig. 1 ). Specific non-polar, unstrained C–H and C–C bonds are cleaved and exchanged in a formal sense. Of note is that the whole transformation is energetically uphill ( vide infra ) and atom-economical. The overall driving force ultimately derives from light. The process can also be extended to the stereoselective synthesis of metacyclophanes 4 possessing planar chirality. 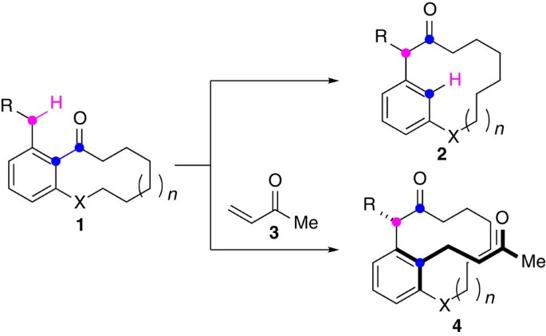Figure 1: Ring expansion reactions. Conversion of orthocyclophanes1to metacyclophanes2and4. Figure 1: Ring expansion reactions. Conversion of orthocyclophanes 1 to metacyclophanes 2 and 4 . Full size image Ring expansion of orthocyclophane 1a to metacyclophane 2a Initially, a THF solution of orthocyclophane 1a (0.02 M) in a Pyrex tube was irradiated with UV light (270–350 nm) for 13 h ( Fig. 2a ). Photocyclization [39] , [40] , [41] took place to afford benzocyclobutenol (±)-5a in 92% isolated yield. Subsequently, the benzocyclobutenol (±)-5a was treated with a catalytic amount of [Rh(OH)(cod)] 2 at 60 °C in MeOH for 5 h. The benzocyclobutene ring was opened with site-selective cleavage of the C( sp 2 )–C( sp 3 ) bond [42] , [43] , [44] , [45] to afford [9]metacyclophane 2a in 72% isolated yield. The 1 H NMR of 2a shows only one singlet peak for the benzylic protons of the ansa chain ( δ 3.67 ( s , 2H)), suggesting that the benzene ring flips up and down freely across the ansa chain. 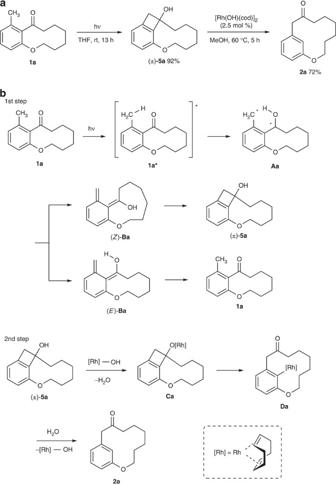Figure 2: Ring expansion of 1a to 2a. (a) Reaction scheme. (b) Plausible mechanism. Figure 2: Ring expansion of 1a to 2a. ( a ) Reaction scheme. ( b ) Plausible mechanism. Full size image A two-step mechanistic sequence for the ring expansion is shown in Fig. 2b . The first step is a photo-induced ring closing reaction ( Fig. 2b , top). According to the mechanism originally proposed by Wagner et al. [41] , the ketone 1a is electronically excited and the excited carbonyl group acts as an oxyl radical to site-specifically abstract the benzylic hydrogen [46] , [47] . The resulting 1,4-biradical species Aa , having an o -phenylene linker, spontaneously generates an isomeric mixture of the o -quinodimethanes ( E )- and ( Z ) -Ba [48] . The ( Z )-isomer having an outward-oriented hydroxy group undergoes a 4π-electrocyclic ring closure to form benzocyclobutenol (±)-5a . On the other hand, the ( E )-isomer having an inward-oriented hydroxy group undergoes facile 1,5-proton shift to regenerate 1a rather than the ring closure. The second step is a ring-opening reaction promoted by the rhodium hydroxide complex ( Fig. 2b , bottom). The hydroxy group of (±)-5a is exchanged onto the rhodium hydroxide to generate rhodium benzocyclobutenolate Ca , in which the benzene ring likely π-coordinates to rhodium [49] . Next follows β-carbon elimination, for which the π-coordination facilitates site-selective cleavage of the C(ipso)–C( sp 3 ) bond to furnish arylrhodium Da . Finally, protonation produces [9]metacyclophane 2a . In order to assess the thermodynamics of this sequential process, DFT calculations were performed at the B3LYP/6-31 G(d) level (Gas phase at 1 atm, 298 K) ( Supplementary Fig. 1 ). The results suggest that (±)-5a and 2a are thermodynamically less stable than 1a by ca. 32.3 and 3.8 kcal mol −1 , respectively. The irreversible formation of highly energetic intermediate (±)-5a by the first photocyclization process makes it possible to drive the energetically uphill transformation from the reactant 1a to its more strained constitutional isomer 2a . Synthesis of planar-chiral cyclophanes 4 We next tried to utilize the arylrhodium intermediate D for the subsequent C–C bond formation, aiming at the synthesis of metacyclophanes having stable planar chirality. Thus, the racemic benzocyclobutenol (±)-5a was treated with a rhodium catalyst in the presence of methyl vinyl ketone ( 3 , 10 equiv.) in toluene at room temperature for 10 h ( Fig. 3 ). The reaction furnished [9]metacyclophane 4a (69% isolated yield) that successfully incorporated 3 at the arene carbon between the 1,3-ansa chain. The 1 H NMR of 4a shows the two distinctly coupled doublets at δ 3.44 ( d , J =14.6 Hz, 1 H) and δ 3.95 ( d , J =14.6 Hz, 1 H), indicating the inequivalency of the two benzylic protons of the ansa chain. The chiral HPLC analysis of the 4a exhibited two peaks of equal intensities in consistence with a racemic mixture of two enantiomers. We assume that the sterics of the middle substituent prohibit the flipping of the benzene ring and give rise to stable planar chirality. 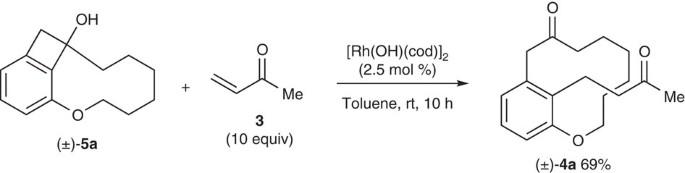Figure 3: Planar chiral derivatives. Rhodium-catalysed reaction of(±)-5awith3. Figure 3: Planar chiral derivatives. Rhodium-catalysed reaction of (±)-5a with 3 . Full size image Next, our interest was directed to the stereochemical course of the ring opening/addition process, during which central chirality of benzocyclobutenol 5a disappeared and planar chirality was generated with 4a . The racemic mixture of benzocyclobutenol (±)-5a was successfully separated by preparative chiral HPLC to the two enantiomers (+)- and (–)- 5a . The reaction of (+)- 5a (>99:1 enantiomeric ratio (er)) with 3 in the presence of the achiral [Rh(OH)(cod)] 2 catalyst afforded (+)- 4a in 72% yield ( Fig. 4 ). A chiral HPLC analysis showed that the enantiomeric purity was retained (>99:1 er). This result assured the stereochemical integrity during the transfer of central chirality of 5a to planar chirality of 4a (ref. 50 ), letting us examine the stereospecificity of chiral transfer in more detail. Thus, the two-step ring expansion of orthocyclophane 1b to metacyclophane (±)-4b was carried out ( Fig. 5a ). 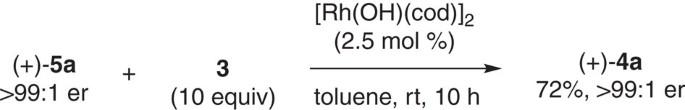Figure 4: Enantiopure starting materials. Synthesis of chiral cyclophane (+)-4a. Figure 4: Enantiopure starting materials. Synthesis of chiral cyclophane (+)- 4a . 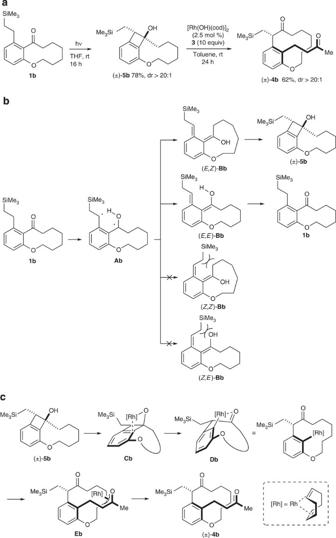Figure 5: Synthesis of cyclophane (±)-4b from 1b. (a) Reaction scheme. (b) Reaction pathway from1bto(±)-5b. (c) Reaction pathway from(±)-5bfrom4b. Full size image Figure 5: Synthesis of cyclophane (±)-4b from 1b. ( a ) Reaction scheme. ( b ) Reaction pathway from 1b to (±)-5b . ( c ) Reaction pathway from (±)-5b from 4b . Full size image The first photocyclization of 1b afforded benzocyclobutenol (±)-5b as a single diastereomer (78% isolated yield). It was determined by NOE analysis that the hydroxy group was trans to the (trimethylsilyl)methyl substituent. Subsequent treatment of (±)-5b with the rhodium catalyst in the presence of 3 (10 equiv) in toluene at room temperature for 24 h furnished [9]metacyclophane (±)-4b in 62% isolated yield, again as a single diastereomer. No other diastereomer was detected in the crude reaction mixture. The (trimethylsilyl)methyl substituent and the C–C bond newly formed between the arene and 3 were assigned as trans to each other by a series of NMR analyses ( 1 H, 13 C, DEPT, COSY, HMQC, HMBC and NOESY). The plausible explanation for the diastereoselectivity observed in the first photocyclization step is shown in Fig. 5b (ref. 41 ). Although the 1,4-biradical species Ab generated from 1b potentially gives rise to four stereoisomers ( E , Z )- Bb , ( E , E )- Bb , ( Z , Z )- Bb and ( Z , E )- Bb , the formation of ( Z , Z )- Bb and ( Z , E )- Bb is disfavoured because of steric repulsion arising between the trimethylsilylmethyl group and the ansa chain. As with the cases of ( Z )- and ( E )- Ba in Fig. 2 , the quinodimethane ( E , Z )- Bb having the outward-oriented hydroxy group undergoes thermal conrotatory electrocyclic ring closure to form trans -benzocyclobutenol (±)-5b diastereoselectively, whereas the isomer ( E , E )- Bb bearing an inward-oriented hydroxy group immediately reverts to the starting ketone 1b via facile 1,5-proton shift. The second ring-opening step occurs with central-to-planar chirality transfer [50] ( Fig. 5c ). The benzene ring of the deprotonated intermediate Cb coordinates to rhodium to facilitate site-selective migration of the ipso sp 2 carbon onto rhodium. For the ipso carbon to migrate onto rhodium, the benzene ring flips up toward rhodium. Accordingly, the developing C–Rh linkage is trans to the (trimethylsilyl)methyl substituent with respect to the newly expanded ansa chain. The rhodium with the COD ligand on it is sterically bulky enough to prohibit the ring flipping across the ansa chain. The intermediate Db then undergoes conjugate addition to 3 with retention of the upward orientation of the C–Rh linkage, producing (±)-4b stereoselectively. Stereoselective production of (±)-4b from (±)-5b provides a strong support for the validity of the stereospecificity of β-carbon elimination. Nonetheless, there remains a possibility that the formation of the diastereomer (±)-4b is favoured over that of the other diastereomer simply due to thermodynamic or kinetic reasons, rather than a mechanistic consequence. In order to examine this possibility, we next carried out the rhodium-catalysed reactions of diastereomeric benzocyclobutenols, trans - and cis -(±)- 5c , which were prepared from 1c having an additional methyl group next to the trimethylsilylethyl substituent ( Fig. 6a ). 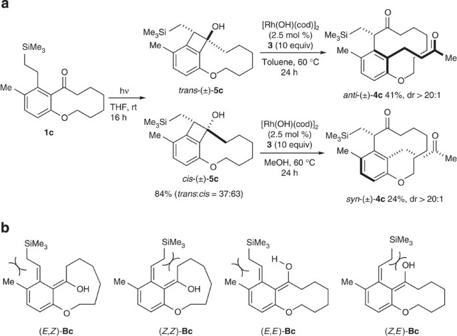Figure 6: Synthesis of cyclophane (±)-4c from 1c. (a) Reaction Scheme. (b) Structures of possible quinodimethane intermediatesB. Figure 6: Synthesis of cyclophane (±)-4c from 1c. ( a ) Reaction Scheme. ( b ) Structures of possible quinodimethane intermediates B . Full size image The result of the first photocyclization step of 1c contrasted with that of 1b , affording a diastereomer mixture of trans- (±)- 5c and cis -(±)- 5c (84%, 37:63). While there are four stereoisomers possibly generated from the biradical intermediate ( Fig. 6b ), those having an inward-oriented hydroxy group immediately revert to the starting 1c , as with the case of 1b . Unlike with 1b , however, the stereoisomer ( E , Z )- Bc is not favoured any more than ( Z , Z )- Bc due to the steric repulsion arising between the (trimethylsilyl)methyl group and the added methyl group. Accordingly, conrotatory ring closure occurs with both ( E , Z )- Bc and ( Z , Z )- Bc to give a mixture of trans -(±)- 5c and cis -(±)- 5c , respectively. Then, the two diastereomers trans -(±)- 5c and cis -(±)- 5c were separated by chromatography on silica gel, and each isolated diastereomer was subjected to the second ring-opening reaction. The diastereomer trans -(±)- 5c with its hydroxy group directing upward (that is, trans to the (trimethylsilyl)methyl substituent) selectively furnished the product anti -(±)-4c with the newly formed C–C bond directing upward (that is, trans to the(trimethylsilyl)methyl substituent). On the other hand, the other diastereomer cis -(±)- 5c with its hydroxy group directing downward (that is, cis to the (trimethylsilyl)methyl substituent) selectively furnished the product syn -(±)- 4c with the newly formed C–C bond directing downward (that is, cis to the (trimethylsilyl)methyl substituent). Thus, a clear stereospecific relationship was observed with the pair of diastereomers trans -(±)- 5c and cis -(±)- 5c to establish that β-aryl elimination occurs in a stereospecific fashion. Various orthocyclophanes 1 were successfully expanded into metacyclophanes (±)- 4 via (±)- 5 in a stereospecific manner by sequential action of light and rhodium ( Table 1 ). The carbocyclic ketone 1g was also transformed to (±)-4g diastereoselectively, although the photocyclization suffered from the formation of the isomeric benzocyclobutenol (±)- 6 (entry 5). The ring expansion of 11-membered cyclic ketone 1h produced (±)-4h , which also possessed planar chirality stable at room temperature (entry 6). Table 1 Ring Expansion of 1 * . Full size table We have described a ring-expanding pathway from orthocyclophanes 1 to their constitutional isomers, metacyclophanes 2 by means of the sequential action of light and rhodium. Formally, the specific non-strained C–H and C–C bonds are cleaved and rearranged to form a product that is energetically uphill. The energy uptake during photocyclization step drives the transformation forward. Furthermore, the present reaction is successfully extended to the synthesis of metacyclophanes possessing planar chirality to demonstrate that stereospecific chirality transfer takes place during the process of rhodium-catalysed C–C bond cleavage. General All reactions were carried out under an argon atmosphere unless otherwise noted. Photoreactions were carried out using RPR-100 photoreactor (Rayonet). Gel permeation chromatography (GPC) was carried out with a Japan Analytical Industry LC-9204. Flash column chromatography was performed with silica gel 60 N (Kanto). Preparative thin-layer chromatography was performed on silica gel plates with PF254 indicator (Merck). Infrared spectra were recorded on a Shimadzu FTIR DR-8000 spectrometer. 1 H and 13 C NMR spectra were recorded on a Varian Mercury vx400 ( 1 H at 400 MHz and 13 C at 100 MHz) spectrometer using CDCl 3 ( 1 H, δ =7.26) and CDCl 3 ( 13 C, δ =77.0) as an internal standard unless otherwise noted. High-resolution mass spectra were recorded on a Thermofisher EXACTIVE (APCI). Optical rotation was measured by a JASCO P-1020 polarimeter with a sodium lamp. HPLC analysis was performed by 4.6 × 250 mm column. For NMR spectra of compounds 1 , 2 , 4 , 5 and HPLC traces of 4a and 5a , please see Supplementary Figs 2–60 . Materials Preparation of orthocyclophanes 1 is described in Supplementary Methods . Anhydrous THF was purchased from Kanto Chemical Co. Anhydrous MeOH was purchased from Wako Pure Chemical Industries. Toluene was distilled from sodium/benzophenone ketyl. Methyl vinyl ketone was distilled from K 2 CO 3 and CaCl 2 prior to use. Photocyclization of orthocyclophane 1a An anhydrous THF solution (5.0 ml) of 1a (21.8 mg, 0.10 mmol) in a Pyrex tube was irradiated under UV light (270–350 nm). After 15 h, the mixture was evaporated. The residue was purified by preparative thin-layer chromatography on silica gel (hexane:AcOEt=5:1) to afford (±)-5a (20.0 mg, 0.092 mmol, 92%). 1 H NMR: δ =1.12–1.28 ( m , 1H), 1.35–1.64 ( m , 5H), 1.69–1.80 ( m , 1H), 1.83–1.97 ( m , 1H), 2.06–2.19 ( m , 1H), 2.28 ( ddd , J =14.4, 8.0, 1.6 Hz, 1H), 3.13–3.24 (m, 2H), 3.91 ( ddd , J =10.4, 8.0, 2.0 Hz, 1H), 4.57 ( ddd , J =10.4, 6.4, 2.0 Hz, 1H), 6.71 ( dd , J =8.4, 0.4 Hz, 1H), 6.77 ( dd , J =7.2, 0.8 Hz, 1H), 7.23 ( dd , J =8.0, 7.2 Hz, 1H); 13 C NMR: δ =21.4, 24.6, 27.5, 28.9, 38.3, 48.4, 72.6, 80.4, 115.0, 117.0, 130.9, 137.2, 142.5 and 154.3; IR (neat): 3,385, 2,920, 1603, 1,456, 1,273, 1,047 and 775 cm −1 ; HRMS ( m/z ): [M+H] + calcd. for C 14 H 19 O 2 , 219.1380; found, 219.1376. Rhodium-catalysed ring opening of (±)-5a A mixture containing [Rh(OH)(cod)] 2 (1.1 mg, 2.5 μmol, 2.5 mol %) and tricyclic benzocyclobutenol (±)-5a (21.4 mg, 0.10 mmol) in MeOH (0.50 ml) was stirred at 60 °C for 5 h. The reaction mixture was passed through a pad of florisil and eluted with ethyl acetate and evaporated. The residue was purified by preparative thin-layer chromatography on silica gel (Hexane:AcOEt=20:1) to afford metacyclophane 2a (15.7 mg, 0.072 mmol, 72%): 1 H NMR: δ =0.98–1.11 ( m , 2H), 1.33–1.47 ( m , 2H), 1.61–1.79 ( m , 4H), 2.26 ( dd , J =6.0, 6.0 Hz, 2H), 3.67 ( s , 2H), 4.25 ( dd , J =4.8, 4.8 Hz, 2H), 6.66 ( s , 1H), 6.76 ( d , J =7.2 Hz, 1H), 6.78–6.84 (m, 1H), 7.23 ( dd , J =8.0, 8.0 Hz, 1H); 13 C NMR: δ =22.4, 22.7, 24.4, 31.3, 35.8, 50.9, 63.4, 112.1, 116.3, 121.7, 130.4, 135.9, 159.9 and 209.8; IR (neat): 2,922, 1,697, 1,587, 1,161 and 783 cm −1 ; HRMS ( m/z ): [M+H] + calcd. for C 14 H 19 O 2 , 219.1380; found, 219.1377. Synthesis of metacyclophane (±)-4a A mixture containing [Rh(OH)(cod)] 2 (1.2 mg, 2.5 μmol, 2.5 mol %), methyl vinyl ketone 3 (81.6 μl, 1.0 mmol) and (±)-5a (21.8 mg, 0.10 mmol) in toluene (0.50 ml) was stirred at room temperature for 10 h. The reaction mixture was passed through a pad of florisil using ethyl acetate as the eluent, and then the filtrate was evaporated. The residue was purified by preparative thin-layer chromatography on silica gel (Hexane:AcOEt=5:1) to afford (±)-4a (19.9 mg, 0.069 mmol, 69%). 1 H NMR: δ =0.25–0.45 ( m , 1H), 0.51–0.68 ( m , 1H), 0.77–0.98 ( m , 3H), 1.27–1.61 ( m , 3H), 1.93–2.13 ( m , 5H), 2.50 ( ddd , J =17.6, 9.2, 6.4 Hz, 1H), 2.61 ( ddd , J =17.6, 9.2, 5.6 Hz, 1H), 2.88 ( ddd , J =13.6, 8.8, 6.4 Hz, 1H), 3.30 ( ddd , J =14.4, 9.6, 5.6 Hz, 1H), 3.44 ( d , J =14.6 Hz, 1H), 3.95 ( d , J =14.6 Hz, 1H), 4.08 ( ddd , J =12.0, 6.4, 2.4 Hz, 1H), 4.21 ( ddd , J =11.2, 8.8, 2.0 Hz, 1H), 6.87 ( d , J =7.6 Hz, 1H), 6.94 ( d , J =7.6 Hz, 1H), 7.14 ( dd , J =8.0, 7.6 Hz, 1H); 13 C NMR: δ =21.8, 22.0, 22.6, 26.4, 28.6, 29.7, 36.7, 44.6, 50.9, 72.1, 120.3, 125.9, 127.8, 134.2, 134.3, 157.6, 207.6 and 209.3; IR (neat): 2,941, 1,705, 1,454, 1,232, 9,10, 729 cm −1 ; HRMS ( m/z ): [M+H] + calcd. for C 18 H 25 O 3 , 289.1798; found, 289.1792. Synthesis of (+)- 4a The racemic mixture of (±)-5a was separated by chiral preparative HPLC (Daicel CHIRALPAK OZ-H column, hexane: i -PrOH=90:10). [α] 25 D =+74.0 ( c =1.1 × 10 −2 M in CHCl 3 ). A mixture containing [Rh(OH)(cod)] 2 (1.7 mg, 3.8 μmol, 2.5 mol %), methyl vinyl ketone ( 3 , 122.4 mmol, 1.5 mmol) and (+)- 5a (33.7 mg, 0.15 mmol, >99:1 er ) in toluene (0.90 ml) was stirred at room temperature for 10 h. The reaction mixture was passed through a pad of florisil using ethyl acetate as the eluent, and then the filtrate was evaporated. The residue was purified by preparative thin-layer chromatography on silica gel (Hexane:AcOEt=5:1) to afford metacyclophane (+)- 4a (32.0 mg, 0.11 mmol, 72%, >99:1 er ) (Daicel CHIRALPAK IB column, hexane: i -PrOH=90:10, 0.40 ml min −1 , retention times: t 1 =9.322 min, t 2 =11.09 min), [α] 25 D =+68.4 ( c =2.1 × 10 −2 M in CHCl 3 ). Benzocyclobutenol 5b 1 H NMR: δ =0.13 ( s , 9H), 0.81 ( dd , J =14.4, 11.2 Hz, 1H), 1.03 ( dd , J =14.8, 4.0 Hz, 1H), 1.07–1.22 ( m , 1H), 1.35–1.61 ( m , 5H), 1.64–1.78 ( m , 1H), 1.89–2.04 ( m , 2H), 2.17–2.30 ( m , 1H), 2.36 ( br s , 1H), 3.39 ( dd , J =11.2, 4.0 Hz, 1H), 3.82–3.90 ( m , 1H), 4.55 ( ddd , J =10.4, 6.0, 1.6 Hz, 1H), 6.70 ( d , J =8.4 Hz, 1H), 6.78 ( d , J =7.2 Hz, 1H), 7.22 ( dd , J =8.0, 7.2 Hz, 1H); 13 C NMR: δ =−0.8, 16.8, 21.2, 25.4, 27.2, 29.1, 34.1, 55.7, 73.0, 82.7, 114.9, 116.5, 130.9, 136.4, 148.1 and 154.4; IR (neat): 3,331, 2,951, 1,601, 1,464, 1,271, 1,244, 1,005 and 854 cm −1 ; HRMS ( m/z ): [M+Na] + calcd. for C 18 H 28 O 2 SiNa, 327.1751; found, 327.1743. Metacyclophane 4b 1 H NMR: δ =−0.03 ( s , 9H), 0.67–0.82 ( m , 1H), 0.83–1.04 ( m , 3H), 1.11 ( dd , J =14.8, 7.2 Hz, 1H), 1.17–1.50 ( m , 5H), 1.87 ( ddd , J =12.8, 10.0, 8.0 Hz, 1H), 2.11 ( s , 3H), 2.25 ( ddd , J =13.2, 10.0, 3.6 Hz, 1H), 2.46 ( ddd , J =18.0, 10.8, 5.2 Hz, 1H), 2.79 ( ddd , J =17.6, 10.4, 5.6 Hz, 1H), 3.23 ( ddd , J =14.0, 10.4, 5.2 Hz, 1H), 3.41 ( ddd , J =13.6, 10.8, 5.6 Hz, 1H), 4.08 (t, J =7.2 Hz, 1H), 4.13 ( ddd , J =12.0, 12.0, 2.8 Hz, 1H), 4.31 ( ddd , J =11.6, 3.6, 3.6 Hz, 1H), 6.85–6.92 ( m , 2H), 7.12 ( dd , J =8.0, 7.6 Hz, 1H); 13 C NMR: δ =−1.0, 15.5, 20.3, 21.7, 23.0, 26.3, 26.4, 29.8, 37.9, 45.0, 51.6, 70.3, 119.1, 121.7, 126.9, 133.5, 138.4, 155.8, 207.8 and 209.9; IR (neat): 2,947, 1,709, 1,454, 1,242, 980 and 831 cm −1 ; HRMS ( m/z ): [M+H] + calcd. for C 22 H 35 O 3 Si, 375.2350; found, 375.2340. Benzocyclobutenol 5c 5c was obtained as a diastereomer mixture that was separated by preparative thin-layer chromatography on silica gel (hexane:AcOEt=10:1). trans - 5c. 1 H NMR: δ =0.12 ( s , 9H), 0.98 ( dd , J =15.2, 10.4 Hz, 1H), 1.06 ( dd , J =15.6, 3.6 Hz, 1H), 1.10–1.22 ( m , 1H), 1.33–1.60 ( m , 5H), 1.62–1.77 ( m , 1H), 1.86–2.05 ( m , 2H), 2.07–2.40 ( m , 5H), 3.41 ( dd , J =10.8, 3.6 Hz, 1H), 3.76–3.87 ( m , 1H), 4.52 ( ddd , J =10.8, 6.0, 1.6 Hz, 1H), 6.61 ( d , J =8.0 Hz, 1H), 6.97 ( d , J =8.0 Hz, 1H); 13 C NMR: δ =−0.8, 15.8, 16.2, 21.5, 25.6, 27.1, 29.0, 34.3, 54.9, 73.1, 82.2, 114.9, 126.2, 131.6, 135.7, 145.8 and 152.3; IR (neat): 3,423, 2,928, 1,618, 1,493, 1,246, 1,020 and 837 cm −1 ; HRMS ( m/z ): [M+Na] + calcd. for C 19 H 30 O 2 SiNa, 341.1907; found 341.1899. cis - 5c . 1 H NMR: δ =−0.09 ( s , 9H), 0.88–1.05 ( m , 2H), 1.10–1.29 ( m , 1H), 1.33–1.60 ( m , 5H), 1.62–1.78 ( m , 1H), 1.82–2.02 ( m , 2H), 2.09–2.29 ( m , 5H), 3.33 ( dd , J =10.0, 4.4 Hz, 1H), 3.84 ( ddd , J =10.4, 8.8, 1.6 Hz, 1H), 4.53 ( ddd , J =10.8, 6.4, 2.0 Hz, 1H), 6.61 ( d , J =8.4 Hz, 1H), 6.97 ( d , J =8.4 Hz, 1H); 13 C NMR: δ =−0.8, 16.2, 16.4, 21.8, 25.3, 27.3, 28.9, 38.7, 52.4, 73.0, 81.6, 115.4, 126.0, 131.6, 135.9, 147.5 and 152.9; IR (neat): 3,396, 2,926, 1,491, 1,244 and 835 cm −1 ; HRMS ( m/z ): [M+Na] + calcd. for C 19 H 30 O 2 SiNa, 341.1907; found, 341.1902. Metacyclophane anti - 4c The reaction was performed at 60 °C. 1 H NMR: δ =−0.02 ( s , 9H), 0.741.07 ( m , 5H), 1.20–1.45 ( m , 4H), 1.77–1.90 ( m , 2H), 2.12 ( s , 3H), 2.19 ( s , 3H), 2.25 ( ddd , J =12.0, 4.0, 4.0 Hz, 1H), 2.44 ( ddd , J =18.0, 11.2, 4.4 Hz, 1H), 2.76 ( ddd , J =18.0, 11.2, 5.2 Hz, 1H), 3.23 ( ddd , J =14.4, 11.2, 4.4 Hz, 1H), 3.60 ( ddd , J =14.0, 11.6, 5.6 Hz, 1H), 4.10–4.27 ( m , 3H), 6.83 ( d , J =8.4 Hz, 1H), 6.90 ( d , J =8.0 Hz, 1H); 13 C NMR: δ =−1.3, 15.7, 20.6, 20.7, 22.5, 26.4, 26.6, 29.7, 29.8, 41.1, 45.3, 50.7, 71.0, 119.4, 130.5, 132.9, 134.1, 136.9, 153.6, 207.8 and 209.0; IR (neat): 2,930, 1,697, 1,450, 1,248 and 837 cm −1 ; HRMS ( m/z ): [M+H] + calcd. for C 23 H 37 O 3 Si, 389.2506; found, 389.2498. Metacyclophane syn - 4c The reaction was performed at 60 °C in MeOH instead of toluene. 1 H NMR: δ =0.02 ( s , 9H), 0.71–0.86 ( m , 2H), 0.90–1.16 ( m , 2H), 1.16–1.32 ( m , 2H), 1.48–1.85 ( m , 5H), 2.01–2.14 ( m , 4H), 2.34 ( ddd , J =16.4, 11.6, 4.8 Hz, 1H), 2.41 ( s , 3H), 2.55 ( ddd , J =16.0, 11.2, 8.4 Hz, 1H), 2.67 ( ddd , J =13.2, 11.6, 4.8 Hz, 1H), 3.16 ( ddd , J =12.8, 10.8, 4.4 Hz, 1H), 3.81 ( dd , J =8.8, 4.4 Hz, 1H), 3.91 ( ddd , J =12.0, 10.0, 1.2 Hz, 1H), 4.31 ( ddd , J =12.4, 5.6, 2.0 Hz, 1H), 6.87 ( d , J =8.4 Hz, 1H), 7.09 ( d , J =8.4 Hz, 1H); 13 C NMR: δ =−1.0, 16.7, 21.3, 22.0, 22.78, 22.83, 26.6, 29.7, 31.0, 35.8, 45.8, 51.8, 73.9, 119.9, 130.4, 131.3, 135.3, 139.3, 158.5, 207.7 and 209.6; IR (neat): 2,949, 1,711, 1,454, 1,246, 980 and 833 cm −1 ; HRMS ( m/z ): [M+H] + calcd. for C 23 H 37 O 3 Si, 389.2506; found, 389.2499. Benzocyclobutenol 5d 1 H NMR: δ =1.12–1.30 ( m , 1H), 1.38–1.64 ( m , 5H), 1.68–1.80 ( m , 1H), 1.87–2.03 ( m , 1H), 2.05–2.15 ( m , 1H), 2.18–2.32 ( m , 1H), 2.84 ( dd , J =14.0, 10.0 Hz, 1H), 3.13 ( dd , J =14.0, 6.0 Hz, 1H), 3.70 ( dd , J =10.4, 6.4 Hz, 1H), 3.87 ( ddd , J =10.8, 9.6, 1.6 Hz, 1H), 4.57 ( ddd , J =10.4, 5.6, 1.6 Hz, 1H), 6.48 ( d , J =7.2 Hz, 1H), 6.71 ( d , J =8.4 Hz, 1H), 7.16 ( dd , J =8.4, 7.2 Hz, 1H), 7.21–7.27 ( m , 1H), 7.28–7.38 ( m , 4H); 13 C NMR: δ =21.3, 25.3, 27.3, 29.2, 34.0, 35.7, 60.0, 73.1, 82.5, 115.4, 116.8, 126.0, 128.4, 128.8, 130.9, 136.4, 140.3, 146.4 and 154.4; IR (neat): 3,331, 2,918, 1,601, 1,454, 1,273, 1,009 and 702 cm −1 ; HRMS ( m/z ): [M+H] + calcd. for C 21 H 25 O 2 , 309.18549; found, 309.1840. Metacyclophane 4d MeOH was employed as a solvent instead of toluene. 1 H NMR: δ =−0.32–0.15 ( m , 1H), 0.67–0.80 ( m , 1H), 0.84–1.11 ( m , 3H), 1.13–1.43 ( m , 3H), 1.50 ( ddd , J =18.0, 10.8, 4.4 Hz, 1H), 1.81–1.95 ( m , 4H), 2.18–2.38 ( m , 2H), 3.02 ( ddd , J =13.6, 10.8, 4.8 Hz, 1H), 3.21 ( dd , J =14.0, 10.0 Hz, 1H), 3.29–3.44 ( m , 2H), 4.09 ( ddd , J =12.0, 12.0, 2.8 Hz, 1H), 4.20 ( dd , J =9.6, 4.8 Hz, 1H), 4.33 ( ddd , J =11.6, 3.2, 3.2 Hz, 1H), 6.89 ( d , J =7.6 Hz, 1H), 7.03 ( d , J =7.6 Hz, 1H), 7.10–7.24 ( m , 6H); 13 C NMR: δ =20.1, 20.9, 23.0, 25.7, 26.5, 29.7, 34.3, 39.8, 44.6, 58.5, 70.2, 119.5, 121.9, 126.1, 126.8, 128.3, 129.2, 134.6, 135.6, 140.4, 155.2, 207.9 and 209.1; IR (neat): 2,855, 1,715, 1,699, 1,456, 1,038, 978 and 700 cm −1 ; HRMS ( m/z ): [M+H] + calcd. for C 25 H 31 O 3 , 379.2268; found, 379.2256. Benzocyclobutenol 5e 1 H NMR: δ =1.04–1.22 ( m , 1H), 1.33–1.77 ( m , 6H), 1.80–2.14 ( m , 3H), 2.16–2.30 ( m , 1H), 3.43 ( dd , J =9.2, 5.6 Hz, 1H), 3.68 ( t , J =6.8 Hz, 2H), 3.86 ( ddd , J =10.8, 1.6, 1.6 Hz, 1H), 4.51–4.62 ( m , 3H), 6.71 ( d , J =6.4 Hz, 1H), 6.72 ( d , J =5.2 Hz, 1H), 7.20 ( dd , J =8.0, 7.2 Hz, 1H), 7.25–7.40 ( m , 5H); 13 C NMR: δ =21.3, 25.3, 27.2, 29.1, 29.9, 34.1, 56.5, 69.2, 73.0, 73.1, 82.1, 115.2, 116.6, 127.6, 127.7, 128.4, 131.0, 136.4, 138.4, 146.6 and 154.4; IR (neat): 3,393, 2,928, 1,603, 1,454, 1,271, 1,080, 1,026, 743 and 696 cm −1 ; HRMS ( m/z ): [M+H] + calcd. for C 23 H 29 O 3 , 353.2111; found, 353.2100. Metacyclophane 4e MeOH was employed as a solvent instead of toluene. 1 H NMR: δ =−0.29–0.13 ( m , 1H), 0.69–0.82 ( m , 1H), 0.91–1.10 ( m , 3H), 1.15–1.45 ( m , 3H), 1.80–1.92 ( m , 4H), 2.13–2.24 ( m , 1H), 2.30–2.40 ( m , 1H), 2.42–2.67 ( m , 3H), 3.21 ( ddd , J =13.6, 10.0, 5.6 Hz, 1H), 3.49 ( ddd , J =13.6, 10.4, 5.2 Hz, 1H), 3.57 ( t , J =5.6 Hz, 2H), 4.12 ( ddd , J =11.6, 2.4, 2.4 Hz, 1H), 4.27 ( t , J =7.6 Hz, 1H), 4.35 ( ddd , J =11.6, 3.2, 3.2 Hz, 1H), 4.44 ( d , J =11.6 Hz, 1H), 4.48 ( d , J =12.0 Hz, 1H), 6.81 ( d , J =8.0 Hz, 1H), 6.91 ( d , J =8.0 Hz, 1H), 7.14 ( dd , J =8.0, 8.0 Hz, 1H), 7.22–7.28 ( m , 3H), 7.29–7.35 ( m , 2H); 13 C NMR: δ =20.1, 21.6, 23.1, 25.9, 26.4, 27.9, 29.5, 39.2, 45.0, 52.1, 67.9, 70.2, 72.7, 119.4, 121.4, 126.9, 127.3, 127.5, 128.4, 134.5, 136.1, 138.4, 155.5, 208.0 and 209.5; IR (neat): 2,943, 1,705, 1,454, 1,240, 1,099 and 733 cm −1 ; HRMS ( m/z ): [M+H] + calcd. for C 27 H 35 O 4 , 423.2530; found, 423.2519. Benzocyclobutenol 5f 1 H NMR: δ =0.02 ( s , 9H), 0.65 ( ddd , J =14.4, 12.4, 4.4 Hz, 1H), 0.77 ( ddd , J =14.4, 12.8, 4.8 Hz, 1H), 1.07–1.23 ( m , 1H), 1.35–1.60 ( m , 6H), 1.64–1.78 ( m , 2H), 1.86–2.01 ( m , 1H), 2.03–2.12 ( m , 1H), 2.15–2.31 ( m , 1H), 2.48 ( br s , 1H), 3.28 ( dd , J =8.8, 6.0 Hz, 1H), 3.86 ( ddd , J =10.8, 9.6, 1.6 Hz, 1H), 4.55 ( ddd , J =10.4, 5.6, 1.6 Hz, 1H), 6.71 ( d, J =8.4 Hz, 1H), 6.84 ( d, J =7.2 Hz, 1H), 7.22 ( dd , J =8.4, 7.2 Hz, 1H); 13 C NMR: δ =−1.7, 15.6, 21.4, 23.8, 25.3, 27.2, 29.1, 33.7, 62.8, 73.0, 82.3, 115.2, 116.3, 130.8, 136.4, 147.5 and 154.4; IR (neat): 3,385, 2,926, 1,603, 1,456, 1,244 and 833 cm −1 ; HRMS ( m/z ): [M+Na] + calcd. for C 19 H 30 O 2 SiNa, 341.1907; found, 341.1899. Metacyclophane 4f 1 H NMR: δ =0.02 ( s , 9H), 0.42 ( ddd , J =14.0, 13.2, 4.8 Hz, 1H), 0.53 ( ddd , J =14.0, 12.8, 4.4 Hz, 1H), 0.69–1.04 ( m , 4H), 1.18–1.52 ( m , 4H), 1.82–1.96 ( m , 2H), 1.97–2.09 ( m , 1H), 2.11 ( s , 3H), 2.20 ( ddd , J =13.6, 10.0, 4.0 Hz, 1H), 2.47 ( ddd , J =17.2, 10.0, 5.2 Hz, 1H), 2.71 ( ddd , J =17.6, 10.0, 5.2 Hz, 1H), 3.18 ( ddd , J =13.6, 10.0, 5.2 Hz, 1H), 3.43 ( ddd , J =13.6, 10.4, 5.2 Hz, 1H), 3.90 ( dd , J =8.0, 6.4 Hz, 1H), 4.15 ( ddd , J =11.6, 11.6, 2.4 Hz, 1H), 4.30 ( ddd , J =12.0, 3.6, 3.6 Hz, 1H), 6.83 ( d , J =6.8 Hz, 1H), 6.92 ( d , J =7.2 Hz, 1H), 7.16 ( dd , J =8.0, 8.0 Hz, 1H); 13 C NMR: δ =−1.8, 14.4, 20.6, 21.5, 22.1, 23.0, 26.4, 26.6, 29.9, 38.2, 45.2, 59.5, 70.6, 119.4, 121.2, 127.2, 134.7, 136.7, 156.0, 207.9 and 210.3; IR (neat): 2,939, 1,713, 1,692, 1,452, 1,248 and 837 cm −1 ; HRMS ( m/z ): [M+H] + calcd. for C 23 H 37 O 3 Si, 389.2506; found, 389.2495. Benzocyclobutenol 5g 1 H NMR: δ =0.13 ( s , 9H), 0.75–1.02 ( m , 3H), 1.07–1.46 ( m , 6H), 1.48–1.79 ( m , 4H), 1.94 ( ddd , J =14.8, 6.0, 2.8 Hz, 1H), 2.08 ( ddd , J =15.2, 10.8, 5.6 Hz, 1H), 2.65 ( ddd , J =14.0, 4.0, 4.0 Hz, 1H), 2.79 ( ddd , J =13.2, 13.2, 4.0 Hz, 1H), 3.29 ( dd , J =12.0, 3.2 Hz, 1H), 6.96 ( d , J =7.2 Hz, 1H), 7.05 ( d , J =8.0 Hz, 1H), 7.23 ( dd , J =7.6, 7.6 Hz, 1H); 13 C NMR: δ =−0.8, 16.9, 20.2, 20.5, 20.9, 27.2, 27.5, 28.5, 31.5, 55.1, 85.9, 119.9, 127.3, 129.6, 137.3 and 146.8, 147.1; IR (neat): 3,319, 2,926, 1,246 and 849 cm −1 ; HRMS ( m/z ): [M+H] + calcd. for C 19 H 31 O 2 Si, 303.2139; found, 303.2130. Metacyclophane 4g The reaction was performed at 60 °C. 1 H NMR: δ =−0.48–0.36 ( m , 1H), 0.052 ( s , 9H), 0.46–0.57 ( m , 1H), 0.69–0.84 ( m , 3H), 1.13–1.30 ( m , 4H), 1.48–1.56 ( m , 1H), 1.67–1.85 ( m , 3H), 2.09 ( s , 3H), 2.21 ( ddd , J =10.0, 7.6, 2.8 Hz, 1H), 2.38–2.57 ( m , 3H), 3.04 ( ddd , J =9.2, 3.6, 3.6 Hz, 1H), 3.10–3.16 ( m , 2H), 3.99 ( t , J =5.2 Hz, 1H), 7.06 ( dd , J =5.2, 0.8 Hz, 1H), 7.18 ( dd , J =5.2, 4.8 Hz, 1H), 7.25 ( d , J =5.6 Hz, 1H); 13 C NMR: δ =−0.8, 16.6, 22.9, 23.4, 24.7, 25.06, 25.12, 26.5, 29.8, 32.8, 34.0, 45.4, 53.4, 125.4, 127.0, 130.1, 136.8, 139.8, 141.4, 207.5 and 211.5; IR (neat): 2,945, 1,715, 1,697, 1,248 and 837 cm −1 ; HRMS ( m/z ): [M+H] + calcd. for C 23 H 37 O 2 Si, 373.2557; found, 373.2548. Benzocyclobutenol 5h 1 H NMR: δ =0.13 ( s , 9H), 0.80 ( dd , J =14.4, 11.2 Hz, 1H), 1.05 ( dd , J =14.4, 4.0 Hz, 1H), 1.18–1.33 ( m , 1H), 1.39–2.02 ( m , 11H), 2.33 ( br s , 1H), 3.35 ( dd , J =11.2, 4.0 Hz, 1H), 3.89–4.02 ( m , 1H), 4.27–4.38 ( m , 1H), 6.73 ( d , J =8.4 Hz, 1H), 6.77 ( d , J =7.2 Hz, 1H), 7.23 ( dd , J =8.4, 7.2 Hz, 1H); 13 C NMR: δ =−0.7, 16.7, 23.4, 23.6, 26.8, 27.2, 28.0, 33.8, 55.7, 69.1, 82.7, 112.1, 115.9, 130.6, 135.5, 148.7 and 153.0; IR (neat): 3,385, 2,868, 1,593, 1,474, 1,244, 1,038 and 833 cm −1 ; HRMS ( m/z ): [M+Na] + calcd. for C 19 H 30 O 2 SiNa, 341.1907; found, 341.1899. Metacyclophane 4h 1 H NMR: δ =0.06 ( s , 9H), 0.49–0.62 ( m , 1H), 0.69–1.05 ( m , 7H), 1.21–1.38 ( m , 1H), 1.41–1.56 ( m , 2H), 1.58–1.72 ( m , 1H), 1.92 ( ddd , J =13.2, 8.8, 6.4 Hz, 1H), 2.12 ( s , 3H), 2.34 ( ddd , J =13.2, 9.2, 6.0 Hz, 1H), 2.45 ( ddd , J =17.6, 10.8, 5.2 Hz, 1H), 2.79 ( ddd , J =17.6, 10.8, 5.6 Hz, 1H), 3.14 ( ddd , J =13.6, 10.4, 5.2 Hz, 1H), 3.35 ( ddd , J =13.6, 10.8, 5.2 Hz, 1H), 4.04 ( dd , J =8.0, 6.4 Hz, 1H), 4.23 ( ddd , J =12.4, 7.2, 2.8 Hz, 1H), 4.29 ( ddd , J =12.0, 7.2, 2.4 Hz, 1H), 6.88 ( d , J =7.6 Hz, 1H), 6.92 ( d , J =8.4 Hz, 1H), 7.13 ( dd , J =8.0, 8.0 Hz, 1H); 13 C NMR: δ =−1.1, 17.6, 20.9, 23.7, 23.8, 26.4, 26.8, 29.5, 29.8, 38.2, 44.3, 51.0, 71.6, 117.1, 121.9, 127.1, 132.1, 139.0, 157.5, 207.9 and 210.8; IR (neat): 2,932, 1,711, 1,246 and 835 cm −1 ; HRMS ( m/z ): [M+H] + calcd. for C 23 H 37 O 3 Si, 389.2506; found, 389.2494. How to cite this article: Ishida, N. et al. Stereospecific ring expansion from orthocyclophanes with central chirality to metacyclophanes with planar chirality. Nat. Commun. 5:3111 doi: 10.1038/ncomms4111 (2014).